Identification of promiscuous ene-reductase activity by mining structural databases using active site constellations The exploitation of catalytic promiscuity and the application of de novo design have recently opened the access to novel, non-natural enzymatic activities. Here we describe a structural bioinformatic method for predicting catalytic activities of enzymes based on three-dimensional constellations of functional groups in active sites (‘catalophores’). As a proof-of-concept we identify two enzymes with predicted promiscuous ene-reductase activity (reduction of activated C–C double bonds) and compare them with known ene-reductases, that is, members of the Old Yellow Enzyme family. Despite completely different amino acid sequences, overall structures and protein folds, high-resolution crystal structures reveal equivalent binding modes of typical Old Yellow Enzyme substrates and ligands. Biochemical and biocatalytic data show that the two enzymes indeed possess ene-reductase activity and reveal an inverted stereopreference compared with Old Yellow Enzymes for some substrates. This method could thus be a tool for the identification of viable starting points for the development and engineering of novel biocatalysts. Enzymes are increasingly used in biotechnological and biocatalytic processes for the ‘green’ production of chemical compounds [1] and in medical applications [2] . Natural enzymes, however, are generally not fully optimized for these purposes. Consequently, not all chemical reactions potentially interesting for biotechnological applications are represented in the currently available enzyme portfolio. Thus, the identification and design of novel enzyme functionalities is of utmost importance. Current approaches include classic wet-lab screening and protein engineering efforts [3] , as well as bioinformatic techniques. The latter often rely on similarities of amino acid sequences (for example, using BLAST or the Catalytic Site Atlas [4] ) or on the conservation of the overall structures and folds of proteins (for example, using PDBeFold [5] ). These computational approaches are mainly used to identify homologous enzymes. By de novo enzyme design, on the other hand, it has recently been possible to build biocatalysts from scratch [6] , [7] , [8] and these methods were successfully applied to generate a variety of protein functions [9] , [10] . However, the designed enzymes also had some drawbacks, such as modest catalytic efficiency or decreased enzyme stability [9] , [11] . In this context, the reutilization of existing enzymes could be beneficial. It has been observed that some natural enzymes—apart from their original catalytic activity—also catalyse completely unrelated chemical reactions as a side activity, known as ‘catalytic promiscuity’ [12] . Examples include the catalysis of C–C bond formation by hydrolases [13] or the nitroaldolase activity of hydroxynitrile lyases [14] . Catalytic promiscuity is generally also seen as the starting point for the evolution of novel enzyme activities in nature [15] . Thus, it could also be a viable basis for engineering novel enzymes [3] provided that a method for the detection of potential catalytic promiscuity is available. Earlier work on three-dimensional (3D) active site templates and database mining, such as TESS [16] and JESS [17] , has shown the potential of structure-based approaches for predicting catalytic activity. Here we describe a method to identify enzymes with specific active site geometries and thus to predict (promiscuous) activities by screening the Protein Data Bank (PDB) using specific 3D templates, which mimic a ‘minimal’ catalytic active site constellation (‘catalophore’) in the style of the theozyme concept [18] . As a test case for our approach, we choose ene-reductase (Old Yellow Enzyme, OYE) activity, that is, the reduction of activated C–C double bonds. This class of enzymes is structurally and mechanistically very well characterized and the reaction has a high potential in biocatalysis, because it allows the simultaneous introduction of two new stereocentres [19] . We identify two enzymes for which we predict promiscuous ene-reductase activity. These enzymes are compared with known ene-reductases regarding their 3D structures (including substrate binding), their biochemical properties, as well as their biocatalytic substrate scope and stereospecificities. These data clearly show that the two enzymes—despite completely different sequences and folds—share salient features of typical OYEs, especially their ene-reductase activity. This example indicates that search methods using structural active site templates may be useful tools for the identification of viable starting points for the development and engineering of novel biocatalysts. 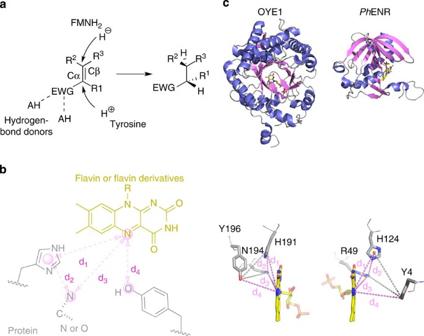Figure 1: Overview of search template and comparison between OYEs and the identified hits. (a) Hydrogenation of activated C–C double bonds catalysed by OYEs (EWG, electron withdrawing group; HA, hydrogen bonding donor). (b) Search template with distance descriptors derived from OYE structures. Amino acids of the protein and the flavin cofactor are represented in grey and yellow, respectively. Spheres represent atoms/pseudo-atoms used for defining distance ranges (d1=7.5–7.9 Å,d2=4.6–5.4 Å,d3=6.1–6.8 Å,d4=5.0–8.9 Å). Undefined bond valences are indicated by dotted lines. (c) Comparison of the overall and active site structures of OYE1 (PDB entry: 1OYB) fromSaccharomyces pastorianusas a typical member of the OYE family and one protomer ofPhENR (PDB entry: 2R6V) identified by the catalophore search. The lower panel shows the positions of the catalytic residues relative to FMN. Distance descriptorsd1–d4are shown as magenta dotted lines. Additional grey dotted lines complete a tetrahedron to better show the approximate mirror symmetry. Database search The database search motif was derived through an analysis of active site constellations in available OYE structures ( Supplementary Table 1 and Supplementary Fig. 1 ). The catalytic site of OYEs harbours a flavin mononucleotide (FMN) cofactor, which donates a hydride to the Cβ atom of the substrate. In addition, it usually comprises a pair of amino acid residues (typically histidine/histidine or asparagine/histidine) that act as H-bonding donors to the electron-withdrawing group of the substrate, and a conserved tyrosine residue (in some cases a cysteine), which is necessary to deliver a proton onto the Cα atom during turnover ( Fig. 1a ). We defined four distances to characterize the relative position of the required functional groups ( Fig. 1b ): from N5 of the flavin cofactor to the geometric centre of the imidazole ring of histidine ( d 1 ), between the histidine and the second hydrogen bonding donor ( d 2 ), between N5 and the second hydrogen bonding donor ( d 3 ) and between N5 and the OH group of the tyrosine ( d 4 ). Figure 1: Overview of search template and comparison between OYEs and the identified hits. ( a ) Hydrogenation of activated C–C double bonds catalysed by OYEs (EWG, electron withdrawing group; HA, hydrogen bonding donor). ( b ) Search template with distance descriptors derived from OYE structures. Amino acids of the protein and the flavin cofactor are represented in grey and yellow, respectively. Spheres represent atoms/pseudo-atoms used for defining distance ranges ( d 1 =7.5–7.9 Å, d 2 =4.6–5.4 Å, d 3 =6.1–6.8 Å, d 4 =5.0–8.9 Å). Undefined bond valences are indicated by dotted lines. ( c ) Comparison of the overall and active site structures of OYE1 (PDB entry: 1OYB) from Saccharomyces pastorianus as a typical member of the OYE family and one protomer of Ph ENR (PDB entry: 2R6V) identified by the catalophore search. The lower panel shows the positions of the catalytic residues relative to FMN. Distance descriptors d 1 – d 4 are shown as magenta dotted lines. Additional grey dotted lines complete a tetrahedron to better show the approximate mirror symmetry. Full size image This motif was then applied in searches in the commercial Relibase+ database [20] . In addition, we implemented an in-house database of protein structures and a script-based search environment using the programme YASARA Structure [21] . 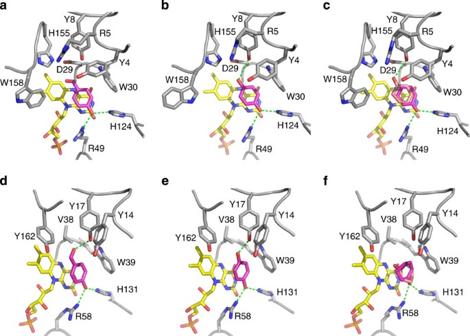Figure 2: X-ray crystal structures of ligand complexes ofPhENR andTtENR. Complexes ofPhENR withp-hydroxybenzaldehyde (a), 1,4-hydroquinone (b) and 2-cyclohexen-1-one (c). Complexes ofTtENR withp-hydroxybenzaldehyde (d), 1,4-hydroquinone (e) and 2-cyclohexen-1-one (f). Amino acid residues are shown in grey, the flavin cofactor in yellow and the bound ligands in magenta. The second, alternate binding mode of 2-cyclohexen-1-one is shown in pink. Hydrogen bonding interactions are depicted as green, dashed lines. The figure was prepared using PyMOL (Schrodinger Inc.). Searches using both database platforms yielded mostly equivalent lists of hits, which not surprisingly contained mainly OYE structures ( Supplementary Table 2 ). The latter were excluded based on sequence similarity as well as on the occurrence of OYE-specific sequence patterns [22] . Two oxidoreductases (PDB entries: 2I0K and 3FBS) were discarded, because the tyrosine residue was located behind the flavin (relative to the other components of the catalophore) and would therefore be unable to act as the proton donor. A flavocytochrome C (PDB entry: 1JRZ) was discarded because of the additional haem cofactor bound to this protein. The two remaining hits, annotated as ‘putative styrene monooxygenase reductase component’ (PDB entries: 1USC and 1USF) from Thermus thermophilus (subsequently named Tt ENR) and as ‘FMN-binding protein’ (PDB entry: 2R6V) from Pyrococcus horikoshii (subsequently named Ph ENR), were further analysed. These two enzymes from extremophiles are homodimers showing a split barrel-like fold [23] , [24] with anti-parallel β-sheets and with one, non-covalently bound FMN molecule per subunit ( Fig. 1c ). This fold is completely different to the (α,β) 8 - or TIM-barrel fold of OYEs. Despite the different fold types, protein sizes and the overall low sequence identities of <10%, both groups of enzymes exhibit very similar arrangements of active site functional groups. Interestingly, however, the active site constellations in Ph ENR and Tt ENR show approximate mirror symmetry to OYE structures ( Fig. 1c ) with the re -face of the isoalloxazine ring (instead of the si -face) being accessible to the substrate, indicating an inverted stereochemical preference [25] of the two enzymes compared with OYEs. X-ray crystallography We determined X-ray crystal structures of ligand complexes of Ph ENR and Tt ENR to analyse the respective binding modes in comparison with OYEs. Although both enzymes crystallized easily and fast, obtaining structures of ligand complexes by soaking and co-crystallization experiments turned out to be more difficult. 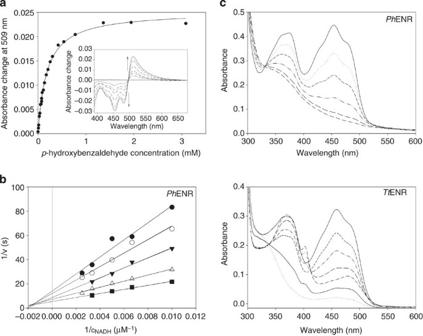Figure 3: Biochemical and spectroscopic analysis. (a) Difference titration ofTtENR withp-hydroxybenzaldehyde. The determinedKdvalue was 25 μM. The insert shows the difference ultraviolet–visible spectra. (b) Double-reciprocal plot of initial rate measurements withPhENR as a function of NADH at 20 (filled circles), 30 (open circles), 50 (filled triangles), 90 (open triangles) and 150 (filled squares) μM of 1,4-benzoquinone. (c) Ultraviolet–visible spectra of anaerobic photoreduction ofPhENR (upper panel) andTtENR (lower panel), where the peak at 402 nm indicates the presence of the red radical species. We managed, however, to obtain diffracting crystals soaked with 2-cyclohex-1-enone, p -hydroxybenzaldehyde ( p HB) and 1,4-hydroquinone, and to determine the structures of the corresponding complexes ( Supplementary Table 3 ). When soaking the crystals with these three ligands, a pronounced colour change from yellow to deep orange was observed, already indicating ligand binding in the vicinity of the FMN cofactor. Indeed, clear residual electron density near the isoalloxazine ring of the flavin was observed in all cases ( Supplementary Figs 2 and 3 ). An analysis using the PISA server [26] confirmed that both proteins are present as dimers in the crystal (and very likely to be in solution). The previously deposited structures of both enzymes, which were identified in the database search (PDB entries: 1USC, 1USF and 2R6V), are very similar to the newly determined complex structures. The root-mean-square deviations after superposition were 0.1–0.2 Å for the comparison of the Ph ENR structures with PDB entry 2R6V and 0.2–0.3 Å for the comparison of the Tt ENR structures with PDB entries 1USC and 1USF. p HB is known as a high-affinity ligand of OYEs [27] , [28] and its binding mode has been elucidated for several members of this enzyme family ( Supplementary Fig. 4 ). In Ph ENR and Tt ENR, an equivalent binding mode was observed. Specifically, the phenolate oxygen atom is hydrogen bonded by His-124 and Arg-49 in Ph ENR or by His-131 and Arg-58 in Tt ENR ( Fig. 2a,d ). Structurally, these residues correspond to the conserved His and Asn residues in OYEs (for example, His-191 and Asn-194 in OYE1 from Saccharomyces pastorianus [29] , Supplementary Fig. 4 ), which act as H-bonding donors to the electron-withdrawing group. The aldehyde group of the ligand is H-bonded to Tyr-17 in Tt ENR (again similar to the binding to OYEs), while a clear interaction partner is missing in the active site of Ph ENR. The third important residue in the active site of OYEs is a tyrosine, which is supposed to act as a proton donor. The residues Tyr-4 in Ph ENR and Tyr-14 in Tt ENR ( Fig. 2 ) correspond to this proton donor in OYEs. Figure 2: X-ray crystal structures of ligand complexes of Ph ENR and Tt ENR. Complexes of Ph ENR with p -hydroxybenzaldehyde ( a ), 1,4-hydroquinone ( b ) and 2-cyclohexen-1-one ( c ). Complexes of Tt ENR with p -hydroxybenzaldehyde ( d ), 1,4-hydroquinone ( e ) and 2-cyclohexen-1-one ( f ). Amino acid residues are shown in grey, the flavin cofactor in yellow and the bound ligands in magenta. The second, alternate binding mode of 2-cyclohexen-1-one is shown in pink. Hydrogen bonding interactions are depicted as green, dashed lines. The figure was prepared using PyMOL (Schrodinger Inc.). Full size image The same binding partners and interactions were also observed in the structures of the two complexes with 1,4-hydroquinone, another phenolic ligand of OYEs ( Fig. 2b,e ). In the structures of the complexes with 2-cyclohexene-1-one, on the other hand, we observed two alternate binding modes in both cases ( Fig. 2c,f ). 2-Cyclohexen-1-one is a typical OYE substrate, which is reduced to cyclohexanone. In the first binding mode the carbonyl group is again H-bonded to His-124 and Arg-49 in Ph ENR or to His-131 and Arg-58 in Tt ENR, respectively. In these structures the Cβ atoms of the α,β-unsaturated carbonyl moiety align well with the N5 atom of the flavin cofactor with distances of 3.4 and 4.5 Å. The relative positions of the predicted proton donors (Tyr-4 in Ph ENR and Tyr-14 in Tt ENR), however, appear to be less optimal with 6–7 Å distances between the OH groups of the tyrosine residues and the Cα atom of the potential substrate. In the second, presumably non-productive binding mode, the ligand is flipped by ∼ 180°. In Ph ENR the carbonyl group is then H-bonded to Tyr-8, but it does not form any specific polar interactions in Tt ENR. Biochemical characterization OYE was the first flavin-dependent enzyme isolated from the brewers’ bottom yeast by Warburg and Christian [30] , and since then has been recognized as a paradigm of flavoproteins. Therefore, a large body of biochemical information is available for the yeast enzyme as well as for other members of the OYE family identified in eubacteria, fungi and plants [31] . We were curious to see to what extent Ph ENR and Tt ENR share properties of the yeast enzyme despite the completely different protein fold. Ligand binding We investigated the binding of different potential ligands using ultraviolet–visible spectroscopic titration experiments. As observed in the soaking experiments, addition of p HB to Ph ENR and Tt ENR gave rise to spectral perturbations in the 550 to 750 nm range, indicating the formation of a charge-transfer complex [28] in a concentration-dependent manner ( Fig. 3a ). The resulting dissociation constants ( K d ) of 36 and 25 μM for Ph ENR and Tt ENR, respectively, are higher than for yeast OYE (0.1 μM) [32] but comparable to the Bacillus subtilis homologue YqjM (24 μM) [33] . Furthermore, binding of the OYE model substrate 2-cyclohexen-1-one was demonstrated for both enzymes, but the determined K d -values of 76 and 40 mM for Ph ENR and Tt ENR, respectively, were substantially higher than for yeast OYE (32 μM) [34] . In addition, we found that 1,4-benzoquinone also binds to both enzymes. However, the K d -values (1.8 mM for Ph ENR and 0.58 mM for Tt ENR) were much lower than in the case of 2-cyclohexen-1-one. This finding suggested that quinones may also act as substrates in the oxidative half reaction (oxidation of the enzyme-bound flavin cofactor). Figure 3: Biochemical and spectroscopic analysis. ( a ) Difference titration of Tt ENR with p -hydroxybenzaldehyde. The determined K d value was 25 μM. The insert shows the difference ultraviolet–visible spectra. ( b ) Double-reciprocal plot of initial rate measurements with Ph ENR as a function of NADH at 20 (filled circles), 30 (open circles), 50 (filled triangles), 90 (open triangles) and 150 (filled squares) μM of 1,4-benzoquinone. ( c ) Ultraviolet–visible spectra of anaerobic photoreduction of Ph ENR (upper panel) and Tt ENR (lower panel), where the peak at 402 nm indicates the presence of the red radical species. Full size image Enzyme kinetics We tested the reoxidation of reduced FMN in Ph ENR and Tt ENR by different, typical OYE substrates and by 1,4-benzoquinone using stopped-flow kinetic measurements under anoxic conditions. Indeed, reoxidation of the reduced cofactor in Ph ENR by 1,4-benzoquinone was complete within the dead time of the stopped-flow instrument, which means that the oxidative rate k ox is >1,000 s −1 . 2-Cyclohexen-1-one, on the other hand, reoxidized the enzyme at a rate of k ox =18 s −1 comparable to the rate determined for yeast OYE ( k ox =102 s −1 ) (ref. 34 ). Interestingly, although 2-methyl-2-pentenal did not generate noticeable spectral perturbations in titration experiments (see above), we were able to determine the reoxidation rate ( k ox =48 s −1 ) and the dissociation constant ( K d =1.26 mM) in stopped-flow experiments. Yeast OYE is efficiently reduced by NADPH showing biphasic kinetics for the reduction of the flavin cofactor [35] with rates of 1.18 and 0.3 s −1 . In contrast, reduction of Ph ENR and Tt ENR with NADPH showed monophasic kinetics with reductive rates ( k red ) of 0.06 and 0.15 s −1 , respectively. An analysis of the concentration dependence of the reduction yielded dissociation constants ( K d ) of 114 μM ( Ph ENR) and 17 μM ( Tt ENR). Interestingly, Tt ENR but not Ph ENR was reduced also by NADH with a k red of 0.25 s −1 , but with a markedly higher dissociation constant ( K d =300 μM). Steady-state turnover experiments with Tt ENR using NADPH and dioxygen as substrates yielded turnover rates of k cat =0.36 s −1 and a K M (NADPH) of 50 μM. This implies that the reductive half reaction is rate-limiting for turnover, because the reoxidation of the cofactor in an air-saturated buffer is two orders of magnitude faster ( k ox =57 s −1 ). The presence of 2-cyclohexen-1-one, 2-methyl-2-pentenal, 4-ketoisophorone, 2-methylcyclo-2-pentenone or p HB had no effect on the rate of NADPH or NADH oxidation. However, 1,4-benzoquinone significantly increased the rate of NADPH and NADH oxidation in a concentration-dependent manner, giving rise to a family of intersecting lines ( Fig. 3b ). This is in contrast to the kinetic behaviour of yeast OYE (OYE2 and OYE3), where the reaction proceeds via a ping-pong bi–bi mechanism involving binary complexes [36] . Although the particular concentration dependence ( Fig. 3b ) may be explained by the formation of a ternary complex, based on the structural constraints of the active site (see Fig. 2 ) it appears more likely to be that the leading substrate (NADPH or NADH) binds to the enzyme in a rapid-equilibrium manner [37] . Photoreduction and redox potential To further investigate the redox properties of the two enzymes, we monitored the photoreduction of the FMN cofactor under anoxic conditions. In both cases the cofactor was fully reduced to the hydroquinone species, accompanied by a loss of the absorbance peaks at 450 and 370 nm ( Fig. 3c ). Only in the case of Tt ENR, small traces of the red anionic semiquinone appeared during photoirradation, but this radical species is clearly not stabilized thermodynamically. This behaviour is similar to yeast OYE, where photoreduction also proceeds to the fully reduced species with only a minor occurrence of the red anionic radical [38] . However, the determination of the redox potentials using NADH or NADPH as reducing agents revealed a major difference to yeast OYE. The measured potentials ( Ph ENR: −325/−320 mV; Tt ENR: −322/−317 mV, with NADPH and NADH, respectively) were ∼ 90 mV lower than that of yeast OYE (−230 mV) [38] . Hence, Ph ENR and Tt ENR substantially alter the redox potential of the FMN cofactor (−210 mV in solution) leading to an ∼ 1,000-fold energetic destabilization of the reduced hydroquinone species, that is, the reduced FMN is a much more powerful reducing agent in both cases. Biocatalytic experiments Several typical OYE substrates were tested to assess the substrate scope and the stereospecificity of Ph ENR and Tt ENR ( Table 1 ). The activation of the C–C double bond necessary to be accepted as a substrate appears to be higher compared with OYEs, but it follows the same general trend [19] , [39] . Therefore, α- and/or β-alkylated ketones ( Table 1 6a – 9a ), which are only weak substrates for other ene-reductases, were not accepted by either of the two enzymes or only converted to a very low extent. On the other hand, 2-methyl-2-pentenal and citral ( 3a and 4a ) as well as compounds bearing two activating groups (4-ketoisophorone 2a and N -phenyl-2-methylsuccinimide 5b ) were good substrates. The unsubstituted ketone 2-cyclohexen-1-one ( 1a ) was accepted but at lower conversion rates. In most cases, Ph ENR turned out to be the more efficient biocatalyst of the two enzymes and we even obtained full conversion in the case of 2-methyl-2-pentenal. Table 1 Biocatalytic transformations. Full size table As indicated by the mirror symmetry of the active sites of Ph ENR and Tt ENR compared with typical OYEs ( Fig. 1c ), both enzymes indeed showed an inverted stereopreference for interesting substrates (that is, 4-ketoisophorone 2a and N -phenyl-2-methylsuccinimide 5bb ), thereby yielding the opposite enantiomer of the reduced product. Our crystallographic, biochemical and biocatalytic studies show that the two enzymes Ph ENR and Tt ENR which were discovered through the catalophore approach share—despite a completely different sequence and fold—some salient features of typical OYEs. These common properties include the binding modes of phenolic ligands and substrates, the reduction of activated C–C double bonds and the utilization of NADPH as the preferred reducing agent. However, the data also unveiled some crucial differences, such as an altered substrate spectrum (for example, quinones), a different kinetic mechanism and a drastically more negative redox potential. Interestingly, the measured redox potentials were also significantly more negative than those obtained for typical reductase components of styrene monooxygenases [40] . This suggests that the putative annotation of Tt ENR (see above) might have to be reconsidered. Taken together, Ph ENR and Tt ENR could be described as NADPH-dependent quinone reductases with significant OYE-like side activities. Such apparent catalytic promiscuity was exactly what we set out to detect with our motif-based catalophore approach. Regarding the potential for biocatalytic applications, the two enzymes turned out to be less efficient catalysts than typical OYEs ( Supplementary Table 4 ), although high conversions were observed for more activated substrates ( Table 1 ). The lower conversion of 2-cyclohexen-1-one could be explained by the occurrence of two alternate binding modes (one productive and one possibly non-productive), which were observed in the X-ray crystal structures of the complexes of Ph ENR and Tt ENR ( Fig. 2c,f ). A remarkable result was the computationally predicted and experimentally confirmed inverted stereopreference of Ph ENR and Tt ENR as in the case of 4-ketoisophorone and N -phenyl-2-methylsuccinimide. Although there are several ways known to switch the enantiopreference of ene-reductases (either by substrate- or enzyme-engineering) [41] , [42] , [43] , up to now the ( S )-enantiomers of these compounds were not accessible by asymmetric bioreduction [19] , [39] . The lower conversions obtained with Ph ENR and Tt ENR are not entirely unexpected, given that the reduction of activated double bonds appears to be only a side activity of these enzymes. However, both enzymes could very well serve as starting points, especially for the development and engineering of stereocomplementary ene-reductases. In summary, this successful test case exemplifies the workflow of identifying (promiscuous) enzyme activity starting from mechanistic and structural considerations. It is a legitimate question, whether the required presence of a cofactor in this specific case is challenging the general applicability of the method, because the presence of a flavin derivative in an enzyme might already imply oxidoreductase activity. Technically, the flavin only contributed another set of geometric restraints to the search template. Of course, increasing the number of these restraints decreases the number of hits, which have to be evaluated. From a functional point of view, it is true that a flavin present in the active site increases the chances of the particular enzyme being an oxidoreductase. In fact, however, only few flavo-enzymes actually show ene-reductase activity and there are also examples of non-redox flavo-enzymes [44] . Search methods using 3D catalytic site constellations are independent of annotations, for example, based on sequence and overall structure similarity. In fact, an increasing number of protein structures are deposited in the PDB, for which no functional annotation is available to date. Another benefit of the method lies in the fact that each hit corresponds to a protein, which has previously been expressed and was stable enough for purification and structure determination. We think that this approach can more generally be used to predict catalytic activities based on 3D structures and to identify novel, non-natural or promiscuous enzyme activities. Thus, it provides an alternative for and complement to existing computational search and design methods, as well as classic wet-lab strategies. Database searches Database searches were carried out in December 2011 against Relibase+ (v2.2) [20] and an in-house database of protein structures, both containing roughly 78,000 PDB entries at that time. For the search in the Relibase+ database the Relibase+ 2D/3D Sketcher was used to create the template with distance cut-offs derived from known OYE structures ( Supplementary Table 1 and Supplementary Fig. 5 ). Because of hard-coded time limits of the Relibase+ (v.2.2) search engine, a subset of structures containing flavin or flavin derivatives was defined before the catalophore search. A slightly modified version of the YANACONDA script (available as a Supplementary File ) was executed in the programme YASARA Structure [21] to search for constellations of functional groups in structures stored in our in-house database consisting of protein structures obtained from the PDB. Code required for the database API is removed for easier reading and stand-alone execution. The script was executed against each available database entry on a Linux-based high-performance computing cluster. It starts by loading the first model record of each PDB file into memory for further processing. The distance ranges d 1 – d 4 can be adapted by changing variables d 11 – d 42 in lines 52 to 62. Structures not containing flavin-like cofactors are discarded (lines 65 to 74). Lines 75 to 163 contain the routines for the distance descriptors. If all distance requirements are fulfilled, a scene file containing the identified constellation is produced and saved, as well as a comma-separated values (CSV) file containing the measured distances, residues and residue numbers for further processing. The obtained results were collected using a Structured Query Language (SQL) backend for data storage and analysis. Owing to slightly different database stocks and search algorithms between Relibase+ and the in-house system, PDB entries 3FBS, 3HGO and 2Q3R were not identified as hits in the in-house database system, whereas PDB entry 3KFT was not identified in the Relibase search. Protein expression and purification Ph ENR The plasmid pSpeedET-Pho containing a gene ( GI:14590716 ) from Pyrococcus horikoshii in a pSpeedET vector was provided by the JCSG (Joint Center for Structural Genomics, CA). The vector pSpeedET is based on a modified pBAD-Thio vector (Invitrogen Life Technologies, Carlsbad, CA) with an additional tobacco-etch-virus (TEV) protease cleavage site. Escherichia coli TOP10F’ cells (Invitrogen Life Technologies) transformed with pSpeedET-Pho were grown in lysogeny broth (LB) medium supplemented with kanamycin (50 μg ml −1 ) at 37 °C. Expression of recombinant protein was initiated by addition of 0.02% arabinose to A 600 ∼ 0.8 cultures, and cultivation was continued for 20 h at 25 °C. Tt ENR A gene ( GI:75345313 ) encoding a putative monooxygenase reductase component from Thermus thermophilus was purchased from Epoch Biolabs Inc. (Sugar Land, TX, USA). No codon optimization was performed. The gene was amplified without stop codon by PCR (forward primer: 5′-AATCACATATGAGGTCCTACCGGGCGC-3′, reverse primer: 5′-AATCAAAGCTTCGGCGCAAAGGTCTCCTCG-3′) from the obtained plasmid. The PCR product was ligated into the Nde I/ Hind III restriction site of pET26b(+), thereby fusing it to a carboxy-terminal His-tag. The construct was confirmed by sequencing (LGC Genomics, Berlin, Germany) and transformed into the expression host E. coli BL21 (DE3) Gold (Agilent Technologies-Stratagene, La Jolla, CA). The transformed cells were grown in lysogeny broth (LB) medium supplemented with kanamycin (50 μg ml −1 ) at 37 °C. Expression of recombinant protein was initiated by addition of IPTG (isopropyl-β- D -thiogalactoside; final concentration 0.5 mM) to A 600 ∼ 0.8 cultures and cultivation was continued for 20 h at 25 °C. Expression and solubility was monitored by SDS–PAGE. The harvested cells were resuspended in cold buffer A (20 mM sodium phosphate buffer pH 7.4 containing 0.5 M NaCl and 10 mM imidazole) and disrupted by sonication (6 min, 80% duty cycle, 70% output; Branson Sonifier S-250, Danbury, CT, USA). The suspension was centrifuged for an hour at 50,000 g . The supernatant was filtered through a 0.45-μm syringe filter and incubated with Ni Sepharose 6 Fast Flow (GE Healthcare, Uppsala, Sweden) for 20 min. The Ni Sepharose was then filled into an empty PD-10 column. After washing with 30 mM imidazole, the bound protein was eluted with 300 mM imidazole in buffer A. Fractions were analysed by SDS–PAGE, pooled and concentrated using Vivaspin 20 Centrifugal Filter Units (10,000 Da cut-off; Sartorius) and desalted on PD-10 columns (GE Healthcare) into 100 mM Tris/HCl, pH 7 ( Ph ENR) or into 20 mM Tris/HCl, pH 7 containing 100 mM NaCl ( Tt ENR). The last purification step for both enzymes was performed on the Äkta Avant (GE Healthcare) using a prepacked Superdex 16/60 column. The eluent was 10 mM Tris/HCl (pH 7.0) and 100 mM NaCl, with an isocratic flow rate of 1 ml min −1 . The protein samples were dialysed against 10 mM Tris/HCl pH 7.5, concentrated to 14 ( Ph ENR) and 7 mg ml −1 ( Tt ENR), and stored at −20 °C. X-ray crystallography Initial crystallization trials employing Morpheus and JCSG+ screens (Molecular Dimensions, Newmarket, UK) were set up using an Oryx8 robot (Douglas Instruments, Hungerford, UK). Crystals of Ph ENR were obtained by vapour diffusion at 20 °C in conditions containing PEG 3350 or 6000 (10–20% w/v) as precipitation agent and different salts (50–200 mM magnesium chloride, potassium formate, sodium formate, ammonium formate, magnesium formate). The crystallization drops were prepared by mixing 0.3–0.5 μl of protein solution (14 mg ml −1 ) with an equal volume of the reservoir solution. Initial crystals of Tt ENR were obtained in crystallization screens using the microbatch method. Several conditions from the Morpheus screen yielded diffraction quality crystals, although growth defects were regularly observed. The best diffracting crystals were obtained with conditions containing 12.5% PEG 1000, 12.5% w/v PEG 3350 and 12.5% v/v 2-methyl-2,4-pentanediol. Diffraction data were collected from crystals obtained in acetate buffer pH 4.5, in 0.1 M sodium HEPES/MOPS buffer system pH 7.5 and in 0.1 M Bicine/Trizma base buffer system pH 8.5. Crystals obtained at pH 7.5 were orthorhombic, the monoclinic crystal used for determining the structure of the 2-cyclo-hexen-1-one complex was obtained at pH 8.5. Crystals of Ph ENR and Tt ENR were soaked for at least 5 min and up to 24 h with potential ligands, including 2-cyclopenten-1-one, 2-cyclohexen-1-one, 2-methyl-2-cyclohexen-1-one, 2-methyl-2-cyclopenten-1-one, 3-methyl-2-cyclopenten-1-one, ( E )-2-methylpent-2-enal, 4-ketoisophorone, p HB, 1,4-hydroquinone, NADP + and NAD + . Co-crystallizations trials with putative ligands were set up using the microbatch method and employing the Morpheus screen. All soaking and co-crystallization experiments were performed under aerobic conditions. Diffraction data were collected from flash-cooled crystals (at 100 K) at the synchrotrons ESRF (beamlines ID14-4, wavelengths 1.004 and 0.980 Å, and BM-14, wavelength 0.976 Å) and Elletra (beamline 5.2R, wavelength 1.0 Å). The data were indexed and scaled using the programmes XDS [45] and SCALA [46] . Structures of Ph ENR and Tt ENR were determined by molecular replacement using structures of both proteins deposited in the PDB entries (2R6V and 1USC) as search models. Molecular replacement was performed using the programme Phaser [47] followed by rounds of refinement using Refmac5 (ref. 48 ) interspersed with manual model rebuilding in Coot [49] . The refinement was only continued if clear difference electron density close to the FMN cofactor indicative of a bound ligand was observed after rigid body refinement. In all cases, R free -values [50] were computed from 5% randomly chosen reflections not used for the refinement. Twin refinement, as included in Refmac5, had to be applied for the refinement of the structure of Tt ENR in complex with 2-cyclohexen-1-one (twinning operator h, -k, -l; twinning fraction 0.48). The stereochemical quality of the models was checked using the programme Molprobity [51] . In all structures, more than 97% of the residues had their main-chain torsion angles in the favoured regions of the Ramachandran plot and none in the disallowed regions. Data collection and refinement statistics are summarized in Supplementary Table 3 . Spectrophotometric methods To determine the extinction coefficient of enzyme-bound FMN, SDS was added to a concentration of 2% and the solution was incubated at 80 °C for 5 min to release the cofactor. Ultraviolet–visible absorption spectra were recorded before and after denaturation of the respective enzyme with a photometer (model Specord 200 plus from Analytik Jena AS, Jena, Germany). All measurements were performed in 20 mM Tris-HCl, pH 8.0, using 1 cm quartz cuvettes. Difference titrations were carried out at 25 °C in tandem cuvettes by the addition of the putative binding partner [2-cyclohexen-1-one, 2-methyl-2-pentenal, 4-ketoisophorone (2,6,6-trimethylcyclohex-2-ene-1,4-dione), 2-methylcyclo-2-penten-1-one, p HB, 1,4-benzoquinone] to a 60-μM enzyme solution in the sample cell and to buffer (50 mM Tris-HCl, pH 7.5) in the reference cell. For photoreduction, the protein was diluted in 50 mM Tris-HCl, pH 7.5, containing 1 mM EDTA and catalytic amounts of 5-deazaflavin. Quartz cuvettes were rendered anaerobic in the nitrogen atmosphere of a glove box. Reduction of the flavin cofactor was achieved by illumination of the sample with a 250-W halogen lamp. Spectra from 300 to 600 nm were recorded at 25 °C until no further changes were observed. Next, the cuvette was opened to air and the absorbance spectrum was recorded. Steady state and stopped-flow kinetics Steady-state turnover of the enzymes was determined by monitoring the oxidation of NADPH and NADH in the presence of molecular oxygen as substrate. Initial velocities were measured by monitoring the decrease of absorbance at 340 nm. All reactions were carried out in 50 mM potassium phosphate (pH 7.0) at 75 °C. The reaction mixture contained 2–5 μM of the respective enzyme, and NADPH or NADH in a concentration range of 50–350 μM. The enzyme activity was calculated using an extinction coefficient of 6,220 M −1 cm −1 for NADPH and NADH. Steady-state turnover rates were also measured by monitoring the oxidation of NADPH or NADH in the presence of 1,4-benzoquinone (20–100 μM) and other putative substrates (2-cyclohexen-1-one, 2-methyl-2-pentenal, 4-ketoisophorone, 2-methyl-2-cyclopenten-1-one, p HB). Stopped flow measurements were carried out with a Hi-Tech (SF-61DX2) stopped flow device (TgK Scientific Limited, Bradford-on-Avon, UK) positioned in a glove box from Belle Technology (Weymouth, UK) at 37 °C. Two reactant solutions were joined in single-mixing mode. FMN oxidation and reduction were measured by monitoring changes in A 458 with a KinetaScanT diode array detector (MG-6560, TgK Scientific Limited). Initial rates were calculated by fitting the curves with Specfit 32 (Spectrum Software Associates, Chapel Hill, NC, USA) using a function of two exponentials. The reductive half reaction was carried out by mixing 40 μM enzyme with NADPH or NADH at a concentration of 0.4–10.0 mM in 100 mM Tris-HCl (pH 7.4). Rate constants for the oxidative half reaction were determined by reduction of 40 μM enzyme in 50 mM potassium phosphate (pH 7.0) by the addition of sodium dithionite. Excess sodium dithionite was removed using a Sephadex PD-10 desalting column inside the glove box. After mixing with the respective substrate at various concentrations in the range of 50 μM to 50 mM, or with air-saturated buffer, the reoxidation of the FMN cofactor was monitored. The used buffer was prepared by flushing with nitrogen followed by incubation in the glove box. The enzyme and substrate solutions were prepared by incubation in the anoxic glove box and dilution with the described buffer. Redox potential measurement Redox potentials of Ph ENR and Tt ENR were measured by titration of the oxidized enzyme in an anaerobic cuvette with NADPH or NADH (end concentration between 20 and 120 μM) as described previously [34] . The solutions were supplemented with 5 μM methylviologen. The titration was recorded by following the ultraviolet–visible spectrum. At the chemical equilibrium of the reaction, the redox potential of NADP + /NADPH equals that of the enzyme. The relative amount of reduced and oxidized enzyme was calculated from the absorbance at 458 nm ( Tt ENR) or 453 nm ( Ph ENR), and the relative amount of NADP + and NADPH was calculated from the absorbance at 337 nm ( Tt ENR) or 330 nm ( Ph ENR), the wavelength where the oxidized and reduced form of each enzyme have the same extinction coefficient. The redox potential of the flavin cofactor was calculated according to the Nernst equation. In this equation, E eq represents the redox potential of both couples at the equilibrium, refers to the midpoint redox potential of the enzyme, and refers to the redox potential of NADP + /NADPH, the value of which was taken as −320 mV. The possibility that the enzyme may have different affinities for NADPH and NADP+ might influence the measured value of the redox potential. Therefore, NADH was also used instead of NADPH for titration. Substrates and reference compounds 2-Cyclohexen-1-one 1a , cyclohexanone 1b , ( E )-2-methylpent-2-enal 3a , rac -2-methylpentanal rac -3b , citral (mixture of E/Z-isomers) 4a , rac -citronellal rac - 4b , ( S )-citronellal ( S )- 4b , N -phenyl-2-methylmaleimide 5a , 3-methyl-2-cyclohexen-1-one 7a , rac -3-methylcyclohexan-1-one rac - 7b , 2-methyl-2-cyclopenten-1-one 8a , rac -2-methylcyclopentan-1-one rac - 8b and rac -3-methylcyclopentan-1-one rac - 9b were purchased from Sigma Aldrich (St Louis, MO, USA). 3-Methyl-2-cyclopenten-1-one 9a was purchased from Fluka (Buchs, Switzerland). 4-Ketoisophorone 2a was purchased from ABCR (Karlsruhe, Germany). rac -2-Methylcyclohexan-1-one rac - 6b was purchased from Alfa Aesar (Karlsruhe, Germany). ( R )-Levodione ( R )- 2b was obtained by bioreduction of 4-ketoisophorone using baker’s yeast (62% e.e. ); rac - N -phenyl-2-methylsuccinimide rac - 5b and 2-methyl-2-cyclohexen-1-one 6a were synthesized as previously reported [52] . rac -2,3-Epoxy-1-cyclohexanone rac -1c and rac -2,3-epoxy-3,5,5-trimethyl-1,4-cyclohexanedione rac -2c were synthesized as previously reported [53] . Chemical formulas of substrates and products are shown in Supplementary Fig. 6 . Biocatalytic transformations In a first step, Ph ENR and Tt ENR were screened for the reduction of the C=C bond of 1a , 2a and 3a by adding an aliquot of the enzyme (100 μg ml −1 ) to a 1.5-ml microcentrifuge tube containing Tris-HCl buffer (0.8 ml, 50 mM, pH 7, 8 or 9), the substrate (10 mM) and the reducing agent (NADH or NADPH, 15 mM). In case of 1a and 2a , the major observed reaction was a Weitz–Scheffer epoxidation ( Supplementary Fig. 7 ) most likely to be due to the FMN-hydroperoxy intermediate or possibly due to free H 2 O 2 , which are produced by the reaction of the reduced cofactor with molecular oxygen [53] ( 1a : Tt ENR: <2% 1b , 9–28% 1c ; Ph ENR: <3% 1b , 4–7% 1c ; 2a : Tt ENR: <0% 2b , 29–83% 2c , Ph ENR: <0% 2b , 7–29% 2c ). Compound 3a showed no epoxidation ( Supplementary Table 5 , entries 1–3) and was therefore selected for further optimization of the reaction conditions. In addition, the optimization was carried out in the absence of oxygen ( Supplementary Table 5 , entries 4–15) to suppress any NAD(P)H oxidase reaction. In procedure, an aliquot of the enzyme (100 μg ml −1 ) was added to a 2-ml screw top glass vial containing degassed buffer (0.8 ml, 50 mM either Tris-HCl buffer, pH 7 or 8; or phosphate buffer, pH 6.2, 7, 7.5 or 8), the substrate (10 mM) and the reducing agent (15 mM). The vial was sealed with a Teflon septum and a screw cap with a hole and flushed with 5 ml Ar. Optimal conditions were 50 mM phosphate buffer for Tt ENR and 50 mM Tris-HCl buffer for Ph ENR both at pH 7, as well as NADPH as reducing agent for both enzymes. In both procedures, the mixture was shaken for 24 h at 30 °C and 120 r.p.m. The products were extracted with EtOAc (2 × 0.5 ml) and the combined organic phases were dried over Na 2 SO 4 . Achiral GC was used to determine conversions and chiral GC or HPLC were used to determine the enantiomeric excess. In case of 5a , the substrate was dissolved in DMF (1% final DMF conc.) for all biotransformations. The reaction products were analysed using achiral GC, as well as chiral GC and HPLC. For details see Supplementary Methods . Accession codes: Atomic coordinates and structure factors have been deposited in the Protein Data Bank under accession codes 3ZOC , 3ZOD , 3ZOE , 3ZOF , 3ZOG and 3ZOH . How to cite this article: Steinkellner, G. et al. Identification of promiscuous ene-reductase activity by mining structural databases using active site constellations. Nat. Commun. 5:4150 doi: 10.1038/ncomms5150 (2014).